Dual pathways of tRNA hydroxylation ensure efficient translation by expanding decoding capability In bacterial tRNAs, 5-carboxymethoxyuridine (cmo 5 U) and its derivatives at the first position of the anticodon facilitate non-Watson–Crick base pairing with guanosine and pyrimidines at the third positions of codons, thereby expanding decoding capabilities. However, their biogenesis and physiological roles remained to be investigated. Using reverse genetics and comparative genomics, we identify two factors responsible for 5-hydroxyuridine (ho 5 U) formation, which is the first step of the cmo 5 U synthesis: TrhP (formerly known as YegQ), a peptidase U32 family protein, is involved in prephenate-dependent ho 5 U formation; and TrhO (formerly known as YceA), a rhodanese family protein, catalyzes oxygen-dependent ho 5 U formation and bypasses cmo 5 U biogenesis in a subset of tRNAs under aerobic conditions. E. coli strains lacking both trhP and trhO exhibit a temperature-sensitive phenotype, and decode codons ending in G (GCG and UCG) less efficiently than the wild-type strain. These findings confirm that tRNA hydroxylation ensures efficient decoding during protein synthesis. RNA modifications confer chemical diversity on simple RNA molecules, expanding their functional repertoires. To date, more than 140 species of RNA modifications have been identified in RNA molecules from all domains of life [1] . In protein synthesis, tRNA serves as an adapter molecule to connect codons on mRNA with the corresponding amino acids. After they are transcribed, tRNAs undergo chemical modifications mediated by site-specific tRNA-modifying enzymes. These modifications play critical roles in stabilizing tRNA tertiary structure and fine-tuning the decoding process [2] , [3] . A wide variety of modifications are present at the first (wobble) position of the anticodon in tRNA (position 34). The wobble modification modulates codon recognition, thereby promoting accurate decoding during protein synthesis [3] , [4] . In the original wobble rule [5] , guanosine at the wobble position (G34) base-pairs with U and C at the third letter of the codon, likewise, uridine at the wobble position (U34) base-pairs with A and G at the third letter of the codon. In Mycoplasma species and mitochondria [6] , [7] , [8] , however, U34 recognizes any of the four bases in a family box through a mechanism called four-way wobbling [3] . To decode two codon sets ending in purine (NNR), U34 is frequently modified to 5-methyl-(2-thio)uridine derivatives [xm 5 (s 2 )U]: 5-carboxymethylaminomethyl-(2-thio)uridine [cmnm 5 (s 2 )U] and 5-methylaminomethyl-(2-thio)uridine [mnm 5 (s 2 )U] in bacterial tRNAs, 5-methoxycarbonylmethyl-(2-thio)uridine [mcm 5 (s 2 )U] and its derivatives in eukaryotic cytoplasmic tRNAs, and 5-taurinomethyl-(2-thio)uridine [τm 5 (s 2 )U] in mitochondrial tRNAs 3 . These modifications prevent tRNAs from misreading near-cognate codons ending in pyrimidines (NNY) [9] . In addition, xm 5 (s 2 )U34 plays a critical role in stabilizing U-G wobble pairing at the A-site of the ribosome [10] , [11] . In contrast to xm 5 (s 2 )U-type modifications, 5-hydroxyuridine derivatives (xo 5 U) are present at the wobble positions of tRNAs responsible for NYN family boxes, and serve to expand decoding capacity in most bacterial species (Fig. 1a, b ). To date, four species of xo 5 U modifications have been reported. 5-carboxymethoxyuridine (cmo 5 U, also called uridine-5-oxy acetic acid) and 5-methoxycarbonylmethoxyuridine (mcmo 5 U, also called uridine-5-oxy acetic acid methyl ester) are found in Gram-negative bacteria, including Escherichia coli and Salmonella enterica [2] , [12] . 5-methoxycarbonylmethoxy-2’ O -methyluridine (mcmo 5 Um) was recently detected in E. coli tRNA Ser as a minor modification [13] . In addition, 5-methoxyuridine (mo 5 U) is present in tRNA Thr from Gram-positive bacteria, including Bacillus subtilis [14] . Using mass spectrometry, we revealed that cmo 5 U34 is present as a major wobble modification in tRNA Leu3 and tRNA Val1 , whereas mcmo 5 U34 is primarily present in tRNA Ala1 , tRNA Ser1 , tRNA Pro3 , and tRNA Thr4 in E. coli [13] (Fig. 1b ). The xo 5 U-type modifications facilitate non-Watson–Crick base pairing with guanosine and pyrimidines at the third positions of codons [15] , [16] , [17] , [18] (Fig. 1b ), thereby contributing to expansion of decoding capability. Moreover, the terminal methylation of mcmo 5 U contributes to decoding ability, at least in tRNA Ala1 [13] . Fig. 1 Decoding capacity of tRNAs is expanded by (m)cmo 5 U. a Secondary structure of E. coli tRNA Ala1 with post-transcriptional modifications: 4-thiouridine (s 4 U), dihydrouridine (D), 2’- O -methyluridine (Um), 5-methoxycarbonylmethoxyuridine (mcmo 5 U), 7-methylguanosine (m 7 G), 5-methyluridine (m 5 U), and pseudouridine (Ψ). A pair of gray triangles indicate the RNase T 1 cleavage positions for analysis of RNA fragments containing the wobble position. b Anticodon–codon pairing in six codon boxes decoded by tRNAs bearing cmo 5 U and mcmo 5 U. Each of the three tRNA genes in parenthesis was individually deleted. In the family boxes (four codons specify a single amino acid), many codons are redundantly decoded by two or three isoacceptors (tRNAs charging with the same amino acid). For example, CUU codon is decoded by tRNA Leu2 with GAG anticodon as well as tRNA Leu3 with cmo 5 UAG anticodon. c Scheme of mcmo 5 U biosynthesis in E. coli . First, U34 is hydroxylated by reactions involving unknown enzymes and substrates to form ho 5 U34 in tRNAs responsible for decoding NYN codons. This reaction requires the chorismate biogenesis pathway. CmoA employs prephenate and AdoMet to generate SCM-SAH with the release of phenylpyruvate and water. Then, ho 5 U34 is carboxymethylated by CmoB using SCM-SAH. Finally, tRNAs responsible for decoding NCN codons are further methylated to generate mcmo 5 U by CmoM in the presence of AdoMet Full size image A structural study of cmo 5 U nucleoside in solution revealed that cmo 5 U adopts the C2’- endo ribose pucker conformation, providing mechanistic insight into base pairing with pyrimidines [9] . The crystal structures of codon–anticodon interactions at the ribosomal A-site revealed that the O5 atom of cmo 5 U is involved in an intramolecular hydrogen bond that pre-structures the anticodon loop, enabling cmo 5 U to pair with pyrimidines at the third position of the codon [19] . In addition, cmo 5 U pairs with G in standard Watson–Crick geometry, rather than classical U-G wobble geometry, indicating that keto-to-enol tautomeric conversion of the uracil base is involved in this base pairing interaction [19] . Multistep reactions are involved in the biosynthetic pathway of cmo 5 U and mcmo 5 U in bacterial tRNAs (Fig. 1c ). Three enzymes, CmoA, CmoB, and CmoM, are involved in the second to last step in the pathway. Initially, U34 is hydroxylated to form 5-hydroxyuridine (ho 5 U) in a reaction catalyzed by unidentified factors. Chorismate, an end product of the shikimate pathway, is involved in this step, but the source of the oxygen atom remains unknown [20] . On the other hand, the subsequent steps have been elucidated. In the second step, a unique carboxymethyl donor, S -carboxymethyl- S -adenosyl- l -homocysteine (SCM-SAH, also called Cx-SAM) is synthesized from AdoMet and prephenate in a reaction catalyzed by CmoA [21] , [22] . CmoB then transfers the carboxymethyl group of SCM-SAH to ho 5 U34 to form cmo 5 U34 on tRNA [21] . In four tRNA species (for Ser1, Pro3, Thr4, and Ala1), cmo 5 U is further methylated by CmoM to form mcmo 5 U34 [13] . The terminal methylation of mcmo 5 U in tRNA Pro3 dynamically alters its modification frequency in a growth phase-dependent manner [13] . Hydroxylation of RNA molecules is a major post-transcriptional modification that plays roles in multiple biological contexts. In addition to xo 5 U modification of bacterial tRNAs, RNA hydroxylation is also responsible for the biogenesis and function of eukaryotic RNA modifications. The JmjC domain-containing protein TYW5 is responsible for biogenesis of hydroxywybutosine (OHyW) at position 37 of mammalian tRNA Phe [23] . ALKBH1 catalyzes tRNA hydroxylation to form 5-hydroxymethyl-2’ O -methylcytidine (hm 5 Cm) and 5-formyl-2’ O -methylcytidine (f 5 Cm) in cytoplasmic tRNA Leu , as well as 5-formylcytidine (f 5 C) in mammalian mitochondrial tRNA Met [24] . ALKBH1-knockout cells exhibit respiratory defects, indicating that ALKBH1 is required for efficient mitochondrial activity. Recently, we discovered hydroxy- N 6 -threonylcarbamoyladenosine (ht 6 A) in echinoderm mitochondrial tRNA; [25] this modification alters the genetic code in echinoderm mitochondria. N 6 -methyladenosine (m 6 A) and 1-methyladenosine (m 1 A) are demethylated by ALKBH family proteins via hydroxymethyl formation [26] , [27] . The Tet protein is responsible for forming 5-hydroxymethylcytidine (hm 5 C) in Drosophila mRNAs [28] . All of the hydroxylases, including the JmjC, ALKBH, and Tet families, are Fe(II)- and 2-oxoglutarate (2-OG)-dependent oxygenases that use a molecular oxygen as a substrate for hydroxylation [29] . Recently, we identified RlhA as a factor responsible RNA hydroxylation to form 5-hydroxycytidine (ho 5 C) at position 2501 in E. coli 23S rRNA [30] . RlhA does not have any characteristic motifs conserved among the known RNA oxygenases, but it does belong to a family of proteins bearing the peptidase U32 motif. This finding encouraged us to explore other peptidase U32-containing proteins responsible for hydroxylation of biological molecules. To search for genes responsible for RNA modifications, we developed a method called ribonucleome analysis to screen knockout strains for uncharacterized genes by liquid chromatography–mass spectrometry (LC/MS) [31] . If a target RNA modification is absent in a certain knockout strain, we can identify the gene dedicated to biogenesis of the target RNA modification via reverse genetics. Using this approach, we have discovered dozens of genes responsible for RNA modifications in tRNAs [13] , [23] , [32] , [33] , [34] , [35] , [36] , [37] , [38] , [39] and rRNAs [30] , [40] , [41] . In this study, we apply ribonucleome analysis in conjunction with comparative genomics to identify two genes, trhP and trhO , which are responsible for formation of ho 5 U at the initial step of xo 5 U biogenesis at the wobble position of bacterial tRNAs. TrhP, a peptidase U32 family protein, is involved in prephenate-dependent ho 5 U34 formation. TrhO, a rhodanese family protein, catalyzes oxygen-dependent ho 5 U34 formation under aerobic conditions. These two pathways play redundant roles in ho 5 U34 formation. Double knockout of both enzymes causes a temperature-sensitive phenotype and decreases the efficiency with which codons ending in G (GCG and UCG) were decoded, indicating that ho 5 U34 formation ensures efficient decoding during translation. E. coli yegQ is involved in tRNA hydroxylation We recently reported that RlhA is responsible for ho 5 C formation at position 2501 in E. coli 23S rRNA [30] . RlhA belongs to a family of proteins that contain the peptidase U32 motif. This finding prompted us to speculate that other paralogs of peptidase U32-containing proteins are involved in ho 5 U34 formation in tRNAs. The E. coli genome contains four paralogs of peptidase U32-containing proteins: rlhA , yegQ , yhbU , and yhbV (Supplementary Fig. 1 , Supplementary Data 1 ). We extracted total RNA from each of the respective knockout strains, digested with RNase T 1 , and subjected the digests to capillary LC-nano-ESI-mass spectrometry (RNA-MS) to detect tRNA fragments containing cmo 5 U (shotgun analysis). 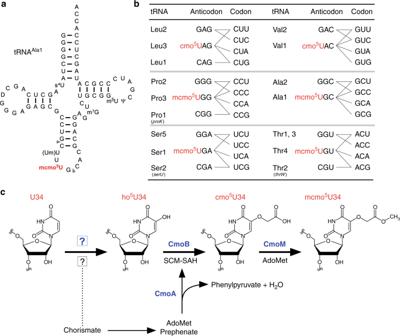Fig. 1 Decoding capacity of tRNAs is expanded by (m)cmo5U.aSecondary structure ofE. colitRNAAla1with post-transcriptional modifications: 4-thiouridine (s4U), dihydrouridine (D), 2’-O-methyluridine (Um), 5-methoxycarbonylmethoxyuridine (mcmo5U), 7-methylguanosine (m7G), 5-methyluridine (m5U), and pseudouridine (Ψ). A pair of gray triangles indicate the RNase T1cleavage positions for analysis of RNA fragments containing the wobble position.bAnticodon–codon pairing in six codon boxes decoded by tRNAs bearing cmo5U and mcmo5U. Each of the three tRNA genes in parenthesis was individually deleted. In the family boxes (four codons specify a single amino acid), many codons are redundantly decoded by two or three isoacceptors (tRNAs charging with the same amino acid). For example, CUU codon is decoded by tRNALeu2with GAG anticodon as well as tRNALeu3with cmo5UAG anticodon.cScheme of mcmo5U biosynthesis inE. coli. First, U34 is hydroxylated by reactions involving unknown enzymes and substrates to form ho5U34 in tRNAs responsible for decoding NYN codons. This reaction requires the chorismate biogenesis pathway. CmoA employs prephenate and AdoMet to generate SCM-SAH with the release of phenylpyruvate and water. Then, ho5U34 is carboxymethylated by CmoB using SCM-SAH. Finally, tRNAs responsible for decoding NCN codons are further methylated to generate mcmo5U by CmoM in the presence of AdoMet RNA fragments were detected as multiply charged negative ions (Supplementary Table 1 ). We clearly detected an anticodon-containing RNA fragment of tRNA Val1 from total RNA of wild-type (WT) E. coli cells (Fig. 2a ). As reported previously [13] , cmo 5 U34 was present as a major wobble modification in this tRNA, whereas little unmodified fragment (U34) was detected. In a knockout strain lacking yegQ (∆ yegQ ), which encodes a peptidase U32-containing protein, cmo 5 U34 frequency decreased markedly, to about 30% of the WT level, and a corresponding fragment containing unmodified U34 appeared, indicating that yegQ is partially responsible for the initial step of cmo 5 U34 formation. We reasoned that other paralogs of peptidase U32-containing proteins might be involved in this process. Accordingly, we constructed a quadruple mutant strain, ∆ yegQ /∆ yhbU /∆ yhbV /∆ rlhA , lacking all paralogs of peptidase U32-containing proteins, and analyzed the RNA fragment of tRNA Val1 . However, the cmo 5 U34-containing fragment persisted in this strain (Fig. 2a ), clearly indicating that another hydroxylation pathway plays a redundant role in the formation of ho 5 U34 in tRNAs. Fig. 2 Identification of trhP responsible for tRNA hydroxylation. a Mass-spectrometric shotgun analysis of total tRNAs in E. coli strains. Extracted ion chromatograms (XICs) show multiply charged negative ions of the anticodon-containing fragments of tRNA Val1 with U34 (upper panels) and cmo 5 U34 (lower) in total tRNAs from wild-type (left), ∆ yegQ (center), and ∆ yegQ /∆ yhbU /∆ yhbV /∆ rlhA strains (right). Sequence, m/z value, and charge state of each fragment are shown on the right. Asterisks indicate nonspecific peaks with the same m/z values. b Mass-spectrometric analysis of the wobble modification in E. coli tRNA Ala1 isolated from WT (left panels) and ∆ yegQ (right) strains. XICs show anticodon-containing fragments of tRNA Ala1 with U34 (top panels), cmo 5 U34 (middle panels), and mcmo 5 U34 (bottom panels). The cleavage sites of RNase T 1 are shown in Fig. 1a . It is assumed that cmo 5 U detected in this tRNA was generated by artificial hydrolysis of mcmo 5 U during tRNA isolation [13] . The black arrowhead indicates a small peak corresponding to the U34-containing fragment detected in the WT. c Modification frequencies of cmo 5 U derivatives at the wobble position of six tRNA species isolated from WT and ∆ yegQ strains. Relative compositions of each modification were calculated from the peak area ratio of mass chromatograms of RNase T 1 digest fragments containing mcmo 5 Um (red), mcmo 5 U (green), cmo 5 U (blue), or U (gray) at the wobble position (Supplementary Fig. 2 ) [13] . Source data are provided as a Source Data file. d Gene organization of a B. subtilis operon containing yrrM , yrrN , and yrrO . Genomic positions in B. subtilis are indicated. The new name for each gene is shown in parenthesis. e Mass-spectrometric shotgun analysis of total tRNAs in B. subtilis strains. XICs are shown of doubly charged negative ions of the anticodon-containing fragments of tRNA Val1a,b with U34 (top panels), ho 5 U34 (middle panels), and mo 5 U34 (bottom panels) in total tRNA from wild-type (leftmost panels), ∆ yrrN (left panels), ∆ yrrO (middle panels), ∆ yrrN /∆ yrrO (right panels), and ∆ yrrM (rightmost panels) strains Full size image To analyze the modification status of each tRNA species in the ∆ yegQ strain, we used the reciprocal circulating chromatography (RCC) method [42] to isolate six tRNA species (tRNA Ala1 , tRNA Leu3 , tRNA Pro3 , tRNA Ser1 , tRNA Thr4 , and tRNA Val1 ) bearing a cmo 5 U34 or mcmo 5 U34 modification from both WT and ∆ yegQ strains. Each tRNA was digested by RNase T 1 and subjected to RNA-MS to analyze the anticodon-containing fragments (Fig. 2b , Supplementary Fig. 2 , Supplementary Table 1 ). Hypomodified fragments were further sequenced by collision-induced dissociation (CID) analysis (Supplementary Fig. 3 ). In tRNA Ala1 , mcmo 5 U34 was present as a major wobble modification in the WT, but its levels were reduced to about 50% (concomitant with appearance of the unmodified fragment) in ∆ yegQ (Fig. 2b ). Similarly, mcmo 5 U34 levels were reduced in tRNA Ser1 and tRNA Thr4 from ∆ yegQ (Fig. 2c , Supplementary Fig. 2 ). The level of cmo 5 U34, a major modification in WT tRNA Val1 , was also reduced about 50% in ∆ yegQ (Fig. 2c , Supplementary Fig. 2 ). By contrast, the levels of cmo 5 U34 of tRNA Leu3 and mcmo 5 U34 of tRNA Pro3 dropped sharply, to less than 5% of WT levels, in the ∆ yegQ strain (Fig. 2c , Supplementary Fig. 2 ). These results indicate that yegQ is involved differently in ho 5 U34 formation in each tRNA. In particular, tRNA Leu3 and tRNA Pro3 are major targets of YegQ. Accordingly, we renamed yegQ as trhP ( tR NA h ydroxylation P ). Biogenesis of mo 5 U34 in Bacillus subtilis Instead of cmo 5 U34 or mcmo 5 U34, B. subtilis uses mo 5 U34 as an xo 5 U-type wobble modification. Upon depletion of intracellular AdoMet, mo 5 U is replaced by ho 5 U [43] , indicating that ho 5 U is the precursor and AdoMet is the methyl donor for mo 5 U formation. We identified two orthologs of trhP in B. subtilis , yrrN and yrrO (Supplementary Fig. 1 , Supplementary Data 1 ), both of which are encoded tandemly in the same operon (Fig. 2d ). YrrO has a peptidase U32 motif and a characteristic C-terminal motif also found in E. coli TrhP, whereas YrrN only has a peptidase U32 motif. We investigated whether these two genes are actually involved in mo 5 U34 formation by shotgun analysis of total RNAs extracted from B. subtilis ∆ yrrN and ∆ yrrO strains. Similar to our observation in the E. coli ∆ trhP strain (Fig. 2a ), mo 5 U34 frequency in tRNA Val1 decreased, and an RNA fragment containing unmodified U34 appeared, in both ∆ yrrN and ∆ yrrO strains (Fig. 2e ), indicating that both yrrN and yrrO were necessary for hydroxylation of U34 to form ho 5 U34 in B. subtilis . Accordingly, we renamed yrrO and yrrN as trhP1 and trhP2 , respectively. To determine whether these two paralogs act redundantly to form ho 5 U34, we constructed the double-deletion strain ∆ trhP1 /∆ trhP2 and analyzed the modification status of tRNA. The same level of mo 5 U34 was detected in this strain as in the single-knockout strains (Fig. 2e ), suggesting that both paralogs are involved in synthesizing about 50% of mo 5 U34 in the cell, and another pathway is required for the remainder, as also observed for formation of cmo 5 U34 in E. coli . We then focused on yrrM , which is encoded within the same operon as trhP1 and trhP2 (Fig. 2d ). B. subtilis YrrM has high sequence similarity to the AdoMet-dependent catechol O -methyltransferase that catalyzes methylation of the hydroxyl group on the aromatic ring, suggesting that this protein is a methyltransferase responsible for mo 5 U34 formation. As expected, mo 5 U34 in tRNA Val1 disappeared and was converted to ho 5 U34 in a ∆ yrrM strain (Fig. 2e ). We then generated recombinant YrrM protein and performed in vitro reconstitution of mo 5 U34 in E. coli tRNA Thr4 containing ho 5 U34, which had been isolated from a ∆ cmoB strain. mo 5 U34 was successfully synthesized in the presence of both YrrM and AdoMet (Supplementary Fig. 4 ). The product was confirmed by CID analysis (Supplementary Fig. 4 ). Taken together, these findings indicate that YrrM is an AdoMet-dependent methyltransferase that converts ho 5 U34 to mo 5 U34 in B. subtilis . During the preparation of this manuscript, B. subtilis yrrM was demonstrated to be a ho 5 U34-methyltransferase and renamed trmR [44] . Alternative pathway for tRNA hydroxylation E. coli trhP and B. subtilis trhP1 / trhP2 are partially involved in the initial step of cmo 5 U34 and mo 5 U34 formation, respectively, indicating the existence of another redundant pathway for ho 5 U34 formation in both species. To search for the gene(s) responsible for this pathway, we used a comparative genomic approach. In bacteria, we found several organisms with cmoA and cmoB homologs, but no trhP homolog (Fig. 3a ). Similarly, some bacteria had a trmR homolog, but no trhP homologs (Fig. 3a ). Given that ho 5 U34 is a common precursor for cmo 5 U34 synthesis mediated by cmoA and cmoB , and mo 5 U34 synthesis mediated by trmR , the bacterial species lacking trhP homologs should have another gene responsible for ho 5 U34 formation independent of the trhP pathway. We identified seven bacterial species with cmoAB or trmR homologs but no trhP or trhP1 / trhP2 homologs (Fig. 3a ). Among 4746 E. coli ORFs, we selected 141 genes (Fig. 3b ) commonly present in all seven species, as well as in B. subtilis . We then narrowed down the list of candidates to seven genes with unknown functions (Fig. 3b ). Among them, a yceA homolog was identified as a strong candidate because its genomic locus is close to that of cmoA in cyanobacteria, and yceA is encoded as a fusion protein with trmR in three bacterial species, Phytophthora sojae , Phytophthora ramorum , and Phaeodatylum tricornutum (Fig. 3b ). To determine whether yceA is responsible for the second pathway of ho 5 U34 formation, we isolated tRNA Val1 from E. coli knockout strains of trhP and yceA , and analyzed the status of wobble modifications. The residual cmo 5 U34 observed in the Δ trhP strain completely disappeared in the double-deletion strain Δ trhP /Δ yceA (Fig. 3c ), indicating that yceA is responsible for the second pathway of ho 5 U34. Hereafter, we refer to yceA as trhO ( tR NA h ydroxylation O ). However, the amount of unmodified U34-containing fragment increased slightly in the single-deletion strain Δ trhO (Fig. 3c ), indicating that the trhP -mediated pathway plays the predominant role in ho 5 U34 formation especially in the absence of trhO . Fig. 3 Identification of trhO responsible for tRNA hydroxylation. a Venn diagram depicts a group of organisms that have cmoAB or trmR homologs but no trhP homologs. Erwinia pyrifoliae , Alcanivorax borkumensis , and Psychrobacter arcticus harbor cmoAB but not trhP ; Pontibacter actiniarum , Ehrlichia canis , and Candidatus phytoplasma harbor trmR but not trhP ; and Dactylococcopsis salina has both cmoAB and trmR but not trhP . b Comparative genomics approach used to narrow down the candidate gene that bypasses ho 5 U34 biogenesis. In Phytophthora sojae , Phytophthora ramorum , and Phaeodatylum tricornutum , yceA and trmR are fused as a single gene. c Mass-spectrometric analysis of the wobble modification in E. coli tRNA Val1 isolated from WT (left panels), ∆ trhP (middle left panels), ∆ yceA (middle right panels), and ∆ trhP /∆ yceA (right panels) strains. XICs show anticodon-containing fragments of tRNA Val1 with U34 (upper panels) and cmo 5 U34 (lower panels). Black arrowheads indicate peaks corresponding to U34-containing fragments detected in the WT and ∆ yceA . Sequence, m/z value, and charge state of each fragment are shown on the right Full size image B. subtilis ybfQ is an ortholog of E. coli trhO . To determine whether ybfQ is involved in the second pathway for ho 5 U34 formation in B. subtilis , we constructed a triple-knockout strain, ∆ trhP1 /∆ trhP2 /∆ ybfQ , and analyzed the status of tRNA wobble modifications. The modified mo 5 U34 in the ∆ trhP1 /∆ trhP2 strain, which was present at about 50% of the WT level, completely disappeared in the triple-deletion strain (Supplementary Fig. 5 ). However, as observed in the E. coli Δ trhO strain, little reduction in the mo 5 U34 level was observed in the single-deletion strain ∆ ybfQ (Supplementary Fig. 5 ). Phylogenetic distribution of trhP and trhO To investigate the phylogenetic distribution of trhP , trhP1 , trhP2 , and trhO , we generated a phylogenetic tree of organisms possessing or lacking each homolog (Supplementary Fig. 6 , Supplementary Data 2 ). trhO orthologs predominated in bacteria and eukaryotes (40%; 232 of 584), whereas trhP orthologs ( yegQ type in Supplementary Fig. 1 ) and trhP1 / trhP2 orthologs (PepU32#5/PepU32#3 in Supplementary Fig. 1 ) were only present in bacteria, and were less widely distributed [14% (84 of 584) and 5% (32 of 584), respectively] (Supplementary Fig. 6 , Supplementary Data 2 ). trhP orthologs were mainly detected in γ- and β-proteobacteria, in addition to some desulfobacteria in δ-proteobacteria. trhP1 / trhP2 orthologs always co-occurred, and were present in phylum Firmicutes and some members of Tenericutes and Cyanobacteria. Given that TrhP1 is a related family with TrhP (Supplementary Fig. 1 ), TrhP1 might have branched out from TrhP, and evolved to require a paralogous protein TrhP2 that might be generated by gene duplication. Supporting this speculation, trhP1 and trhP2 are tandemly encoded in the same operon in B. subtilis (Fig. 2e ). Also, we can explain the reason why trhP orthologs and trhP1 / trhP2 orthologs show a mutually exclusive distribution in bacteria (Supplementary Fig. 6 ). Intriguingly, over half of organisms bearing trhP or trhP1 / trhP2 orthologs also harbor trhO orthologs [49 of 84 (58%) organisms bearing trhP , P = 0.0003 (Fisher’s exact test); 22 of 32 (69%) organisms bearing trhP1 / trhP2 , P = 0.0007 (Fisher’s exact test)] (Supplementary Fig. 7 ). This significant overlap suggests that harboring both pathways for tRNA hydroxylation might help organisms to adapt to two different environments, i.e., aerobic and anaerobic conditions. Phenotypes of E. coli strains lacking tRNA hydroxylation We then measured the growth rate of a series of E. coli knockout strains involved in (m)cmo 5 U34 modifications. No growth reduction was observed in the ∆ cmoM strain, as reported previously [13] (Fig. 4a ), indicating that the terminal methylation of mcmo 5 U34 has little impact on cell growth. A slight increase of doubling time was observed in the ∆ cmoB strain, in which ho 5 U34 accumulated, indicating that the carboxymethyl group of (m)cmo 5 U34 contributes to efficient growth of E. coli cells. Notably, the ∆ trhP /∆ trhO strain grew more slowly than the WT and ∆ cmoB strains, providing a clear evidence for the functional importance of 5-hydroxyl group of (m)cmo 5 U34 in cells. To characterize phenotypic features of the ∆ trhP /∆ trhO strain, we further knocked out tRNA genes responsible for G-ending codons [ serU (tRNA Ser2 ) for the UCG codon, thrW (tRNA Thr2 ) for the ACG codon, and proK (tRNA Pro1 ) for the CCG codon], because these codons are redundantly deciphered by the respective tRNA and the isodecoder with the (m)cmo 5 U34 modification in each codon box. Growth reduction of the ∆ trhP /∆ trhO strain relative to the ∆ cmoB strain was observed upon knockout of serU , thrW , and proK (Fig. 4a ), indicating that the 5-hydroxyl group of (m)cmo 5 U34 plays a critical role in deciphering G-ending codons, especially in the absence of the respective isodecoder. Fig. 4 Phenotypes of E. coli strains lacking tRNA hydroxylation. a Growth rates of E. coli strains with different wobble modifications. Doubling time of WT (mcmo 5 U34 for tRNA Ser1 , tRNA Thr4 , and tRNA Pro3 ), ∆ cmoM (cmo 5 U34), ∆ cmoB (ho 5 U34), and ∆ trhP /∆ trhO (U34) in the presence (left) or the absence of tRNA isodecoders at 37 °C in liquid LB medium: tRNA Ser2 (middle left), tRNA Thr2 (middle right), or tRNA Pro1 (right). Individual data (dot plots) and their means ± SD (bar graph) are presented ( n = 4). * P < 0.01; ** P < 0.001 between two data series (Student’s t -test, one-sided). b Growth of WT, ∆ cmoM , ∆ cmoB , ∆ trhP /∆ trhO , ∆ trhP , and ∆ trhO strains in the absence of tRNA Ser2 (∆ serU ). The expected wobble modification status of each strain is shown on the right. Each strain was serially diluted (1:10), spotted onto LB agar plates, and cultivated for 11 h (30 °C), 8 h (37 °C) or 8 h (42 °C). c Growth of WT, ∆ cmoM , ∆ cmoB , ∆ trhP /∆ trhO , ∆ trhP , and ∆ trhO strains in the absence of tRNA Thr2 (∆ thrW ). The expected wobble modification of each strain is shown on the right. Each strain was serially diluted (1:10), spotted onto M9 minimum agar plates, and cultivated for 31 h (30 °C), 21 h (37 °C), 26 h (40 °C) or 31 h (42 °C). d Schematic of the reporter construct for the dual-luciferase assay, based on the RF2 recoding system. SD, Shine–Dalgarno sequence. Renilla and firefly luciferases were fused with a linker containing the +1 frameshift inductive signal of the RF2 recoding site. The frameshift target site was replaced with a GCG codon for tRNA Ala1 , a UCG codon for tRNA Ser1 , or GG (zero frame) for the control. e Relative pausing activities at the frameshift site with a GCG codon (left), a UCG codon in the presence (middle left) or absence (middle right) of isodecoder tRNA Ser2 , or zero frame (right) were calculated by normalizing Fluc activity vs. Rluc activity and further normalizing against the WT activity in each graph. Individual data and their means ± SD ( n = 4) are presented. * P < 0.01 between two data series (Student’s t -test, two-sided). All source data for Fig. 4 are provided as a Source Data file Full size image Next, we examined the temperature sensitivity of a series of knockout strains involved in (m)cmo 5 U34 modifications. The ∆ trhP /∆ trhO/ ∆ serU strain grew as efficiently as the other strains on LB plates at 30 °C, but slowly at 37˚C and not at all at 42 °C (Fig. 4b ). The growth defect of this strain at 42˚C was restored by introduction of plasmid-encoded trhP (Supplementary Fig. 8 ), indicating that the temperature-sensitive phenotype of this strain can be attributed to hypomodification of tRNA Ser1 . Curiously, the ∆ trhP /∆ serU strain did not exhibit temperature sensitivity, although the frequency of mcmo 5 U34 actually decreased in tRNA Ser1 (Fig. 2c ), indicating that trhO -mediated hydroxylation compensates for the growth defect when the trhP -mediated hydroxylation pathway is impaired. This result highlights the importance of redundant hydroxylation pathways for formation of xo 5 U. Similarly, we observed a severe growth reduction in the ∆ trhP /∆ trhO/ ∆ thrW strain cultivated on M9 minimum plates, even at 40 °C (Fig. 4c ). At 42 °C, this strain was unable to grow, and ∆ cmoB strain exhibited a growth defect. These results clearly demonstrated that the absence of the 5-hydroxyl group of (m)cmo 5 U34 causes a temperature-sensitive phenotype, especially in the absence of the isodecoder responsible for G-ending codons. Decoding properties without tRNA hydroxylation To investigate the functional role of (m)cmo 5 U34 modification in terms of decoding efficiency, we conducted dual-luciferase reporter assays based on the RF2 recoding system [18] , [45] . The reporter constructs consisted of Renilla luciferase (Rluc) fused with firefly luciferase (Fluc) in a +1 frame via a slippery linker derived from the +1 frameshift signal of the RF2 recoding site, so that Fluc expression requires a +1 frameshift at the linker sequence. The UGA codon at the recoding site was substituted with GCG and UCG as test codons to examine their ability to be decoded by tRNA Ala1 and tRNA Ser1 , respectively (Fig. 4d ). We also prepared a control reporter in which the recoding site was replaced with GG (zero frame). These reporters were introduced to a series of E. coli knockout strains lacking genes involved in (m)cmo 5 U34 modifications. The decoding ability of tRNAs with different wobble modifications at each test codon of the frameshift site was negatively correlated with the +1 frameshift activity, measured by Fluc activity, because in this system the +1 frameshift activity is promoted by the hungry A-site. The +1 frameshift activity was calculated by normalizing the Fluc signal against the Rluc signal (F/R value). No difference in F/R value in the control construct (zero frame) was observed in any strains (Fig. 4e ). Using this system, we first measured decoding ability of tRNA Ala1 with different wobble modifications using the GCG-reporter, because in E. coli the GCG codon is solely deciphered by this tRNA (Fig. 1b ). Compared with the WT strain (mcmo 5 U34), we observed clear stimulation of +1 frameshift activity in ∆ cmoM (cmo 5 U34) and ∆ cmoB (ho 5 U34) strains (Fig. 4e ), as reported previously [13] . We also observed a significant increase in +1 frameshift activity in the ∆ trhP /∆ trhO (U34) strain relative to the WT strain (mcmo 5 U34) (Fig. 4e ). These results indicate that tRNA Ala1 gradually loses its decoding ability in response to side-chain shortening of mcmo 5 U34. Next, we measured the decoding ability of tRNA Ser1 with different wobble modifications using the UCG-reporter. In E. coli , UCG codons are redundantly decoded by tRNA Ser1 with the mcmo 5 UGA anticodon and tRNA Ser2 with the CGA anticodon (Fig. 1b ). Relative to the WT strain (mcmo 5 U34), we observed a marked increase in +1 frameshift activity in the ∆ cmoB (ho 5 U34) and ∆ trhP /∆ trhO (U34) strains (Fig. 4e ). Then, we measured the activities of the UCG-reporter in a series of knockout strains in the absence of tRNA Ser2 (∆ serU background). Relative to the ∆ serU strain (mcmo 5 U34), +1 frameshift activity was elevated in both ∆ cmoB /∆ serU (ho 5 U34) and ∆ trhP /∆ trhO /∆ serU (U34) strains (Fig. 4e ). Notably, ∆ trhP /∆ trhO /∆ serU (U34) had significantly higher +1 frameshift activity than ∆ cmoB /∆ serU (ho 5 U34) (Fig. 4e ), indicating that the 5-hydroxyl group of ho 5 U34 on tRNA Ser1 can decode the UCG codon, especially in the absence of isodecoder tRNA Ser2 . Characterization of trhP -mediated tRNA hydroxylation According to our recent study [30] , the shikimate pathway is associated with rlhA -mediated ho 5 C2501 formation in 23S rRNA. A series of genetic studies revealed that prephenate is an essential metabolite for the first step of this modification. Given that TrhP belongs to a family of peptidase U32-containing proteins, we asked whether prephenate is also required for trhP -mediated ho 5 U34 formation. Consistent with this possibility, previous studies reported that the initial step of cmo 5 U34 formation is associated with chorismate biogenesis in E. coli , B. subtilis , and Salmonella typhimurium [20] , [46] . Chorismate is an end product of the shikimate pathway and a common precursor for aromatic amino acids and vitamins in bacteria and plants [47] . Shotgun analyses of E. coli total RNA revealed that cmo 5 U34 formation was significantly impaired in an ∆ aroC strain, in which no chorismate was produced (Supplementary Fig. 9 ). However, ho 5 U34 was still present in this strain because ho 5 U34 was redundantly synthesized by the trhO -mediated pathway. By contrast, as expected, no ho 5 U34 was detected in an ∆ aroC /∆ trhO strain (Supplementary Fig. 10 ). In E. coli , chorismate is converted into five metabolites: isochorismate (catalyzed by the products of entC and menF ), 4-hydroxybenzoate ( ubiC ), 4-amino-4-deoxychorismate ( pabB ), anthranilate ( trpE ), and prephenate ( pheA and tyrA ) (Fig. 5a ). Among these pathways, the ubiC -mediated pathway was excluded because 4-hydroxybenzoate does not restore cmo 5 U34 formation in Salmonella ∆ aroD strain [46] . As observed in the ∆ aroC strain, cmo 5 U34 formation was only impaired in the ∆ pheA /∆ tyrA strain, but not in the ∆ entC /∆ menF , ∆ pabB , and ∆ trpE strains (Supplementary Fig. 9 ), indicating that prephenate or its downstream metabolites are required for ho 5 U34 formation. Fig. 5 Characterization of trhP -mediated tRNA hydroxylation. a A shikimate pathway and related metabolism. Chemical structures of metabolites and the responsible genes (italicized) at each step are shown. Two or three genes at each step indicate a redundant pathway [e.g., prephenate is redundantly synthesized from chorismate mediated by pheA (CM) and tyrA ]. Black or gray arrows represent pathways indispensable or dispensable for trhP -mediated ho 5 U34 formation, respectively (Supplementary Fig. 9 ). White arrows represent pathways not examined in this study. b Genetic complementation of ho 5 U34 formation. Mass-spectrometric shotgun analysis of total tRNAs obtained from the E. coli Δ pheA /Δ tyrA /Δ cmoA /Δ trhO strain transformed with a control plasmid (left panels) or pMW- pheA (CM) (right panels). XICs show multiply charged negative ions of anticodon-containing fragments of tRNA Val1 with U34 (upper panels) and ho 5 U34 (lower panels). Sequence, m/z value, and charge state of each fragment are shown on the right. c Metabolic complementation of ho 5 U34 formation. Mass-spectrometric shotgun analysis of total tRNAs obtained from the E. coli Δ pheA /Δ tyrA /Δ cmoA /Δ trhO strain cultured in the absence (left panels) or presence (right panels) of 1 mM prephenate. XICs show multiply charged negative ions of anticodon-containing fragments of tRNA Val1 with U34 (upper panels) and ho 5 U34 (lower panels). Sequence, m/z value, and charge state of each fragment are shown on the right. d Domain organization of E. coli TrhP, which contains Peptidase_U32 (PF01136) and Peptidase_U32_C (PF16325) domains. Six residues in the Peptidase_U32 domain that are essential for TrhP-mediated hydroxylation are indicated. e Mutation study of trhP . Mass-spectrometric shotgun analysis of total tRNA in the E. coli ∆ trhP strain transformed with plasmid-encoded trhP WT or mutants, as indicated. XICs show multiply charged negative ions of the anticodon-containing fragments of tRNA Val1 with U34 (black lines) and cmo 5 U34 (red lines) in total tRNAs. Sequence, m/z value, and charge state of each fragment are shown on the right Full size image Prephenate is converted to downstream metabolites via three pathways (Fig. 5a ). cmo 5 U34 formation was unchanged in ∆ tyrA and ∆ tyrB strains (Supplementary Fig. 9 ). pheA encodes a fusion of chorismate mutase (CM) and prephenate dehydratase (PDT), which synthesize prephenate and phenylpyruvate, respectively (Fig. 5a ). To dissect these two enzymatic activities, we constructed a pheA variant possessing only the CM activity [pheA(CM)] by introducing an active-site mutation in the PDT domain [48] . To determine whether prephenate is responsible for ho 5 U34 formation, we constructed the quadruple-knockout strain ∆ pheA /∆ tyrA /∆ cmoA /∆ trhO , and then introduced plasmid-encoded pheA(CM), resulting in accumulation of prephenate. ho 5 U34 levels were restored relative to those in a mock transformant (Fig. 5b ). Furthermore, when prephenate was directly added to a culture medium of the quadruple-knockout strain, ho 5 U34 clearly appeared (Fig. 5c ). These results demonstrated that prephenate is required for ho 5 U34 formation. To characterize the peptidase U32 domain of trhP , we mutated each of six conserved residues in this domain (Fig. 5d , Supplementary Fig. 11 ) and examined their activities in vivo by complementation of the ∆ trhP /∆ trhO strain. Shotgun analyses revealed that cmo 5 U34 was fully restored by WT trhP , but not by any of the mutants examined in this study (Fig. 5e ), indicating that the peptidase U32 domain plays a key role in trhP -mediated tRNA hydroxylation. Characterization of trhO -mediated tRNA hydroxylation Given that Fe(II)- and 2-OG-dependent oxygenases use O 2 as a substrate for hydroxylation, we next asked whether molecular oxygen is involved in ho 5 U34 formation. cmo 5 U34 formation is not affected in E. coli cultured under anaerobic conditions [20] , indicating that molecular oxygen is irrelevant to trhP -mediated ho 5 U34 formation. To determine whether O 2 is involved in trhO -mediated ho 5 U34 formation, we cultured the E. coli ∆ trhP strain under aerobic and anaerobic conditions, and then monitored cmo 5 U34 formation by shotgun analysis. Very little cmo 5 U34 was detected in ∆ trhP cells cultured under anaerobic conditions (Fig. 6a ), whereas no reduction in cmo 5 U34 was observed in WT cells (Supplementary Fig. 12 ), implying that O 2 is necessary for trhO -mediated ho 5 U34 formation. We then metabolically labeled ho 5 U34 using 18 O-labeled O 2 . To accumulate ho 5 U34, we cultured the E. coli ∆ trhP /∆ cmoB strain in mixed gas containing 20% 18 O 2 . Total RNA extracted from this culture was digested into nucleosides and subjected to LC/MS. We clearly detected a deprotonated ho 5 U34 nucleoside with molecular mass ( m/z 261) 2 Da greater than that of the naturally occurring nucleoside (Fig. 6b ). CID analysis of the nucleoside revealed that the 18 O atom was present in the base moiety of ho 5 U (Supplementary Fig. 13 ). No oxygens in the uracil base were labeled with 18 O under the 18 O-air condition (Supplementary Fig. 13 ), demonstrating that trhO -mediated tRNA hydroxylation utilizes O 2 as an oxygen atom donor. Fig. 6 Characterization of trhO -mediated tRNA hydroxylation. a trhO -mediated cmo 5 U formation takes place under aerobic conditions. Mass-spectrometric shotgun analysis of total tRNAs obtained from E. coli Δ trhP strain cultured under anaerobic (left panels) or aerobic (right panels) conditions. XICs show negative ions of the anticodon-containing fragments of tRNA Val1 with U34 (upper panels) and cmo 5 U34 (lower panels). Arrowheads indicate target peaks, and asterisks indicate unspecific peaks. b Molecular O 2 is the metabolic source of the hydroxyl group of ho 5 U34 generated by trhO . Mass-spectrometric nucleoside analyses of total RNAs obtained from the E. coli ∆ trhP /∆ cmoB strain cultured in mixed gas with 20% 18 O 2 (left panels) or in normal air (right panels). UV traces at 254 nm (upper panels) and XICs (lower panels) of deprotonated ho 5 U extracted from non-labeled (black line) or [ 18 O]-labeled (red line) cells are shown. c TrhO interacts with tRNA Ala1 specifically. Electrophoretic mobility shift assay (EMSA) was performed to detect direct interaction between recombinant TrhO and tRNA Ala1 (left panels) or tRNA Leu3 (right panels) isolated from E. coli . tRNAs and TrhO were stained with SYBR Safe (upper panels) and Coomassie brilliant blue (lower panels), respectively. TrhO–tRNA complexes are indicated by red traces. Arrowheads indicate unbound intact tRNAs and TrhO. Source data are provided as a Source Data file. d In vitro reconstitution of ho 5 U34 with recombinant TrhO. RNase T 1 digests of E. coli tRNA Ser1 transcripts (10 pmol) incubated with (10 pmol; 1 eq or 100 pmol; 10 eq) or without TrhO are subjected to RNA-MS. XICs show doubly charged negative ions of the anticodon-containing fragments of tRNA transcript with U34 (upper panels) and ho 5 U34 (lower panels). Frequencies of ho 5 U34 are indicated. e Domain organization of E. coli TrhO bearing Rhodanese (PF00581) and Rhodanese_C (PF12368) domains. The CXGGXR motif and six residues mutated in this study are indicated. f Mutation study of trhO . Mass-spectrometric shotgun analysis of total tRNAs in the E. coli Δ trhP /Δ trhO strain transformed with plasmid-encoded trhO WT or mutants, as indicated. XICs show multiply charged negative ions of the anticodon-containing fragments of tRNA Val1 with U34 (black lines) and cmo 5 U34 (red lines) from total tRNA Full size image Next, we generated recombinant E. coli TrhO and subjected it to biochemical characterization. Electrophoretic mobility shift assay (EMSA) revealed that TrhO interacted with tRNA Ala1 , but not with tRNA Leu3 (Fig. 6c ). This result is consistent with our observation that cmo 5 U34 of tRNA Leu3 is mainly synthesized via the trhP -mediated pathway, whereas mcmo 5 U34 of tRNA Ala1 is redundantly synthesized by both the trhP - and trhO -mediated pathways. We then attempted to reconstitute ho 5 U in vitro, and successfully detected ho 5 U on tRNA Ser1 in the presence of recombinant TrhO. When TrhO was present in excess, 75% of the tRNA had ho 5 U (Fig. 6d ). CID analysis of the modified fragment confirmed that ho 5 U was formed at position 34 of the tRNA (Supplementary Fig. 14 ). This result demonstrated that TrhO is an RNA hydroxylase that can form ho 5 U34 on tRNA by utilizing O 2 as an oxygen donor. TrhO is a rhodanese family protein characterized by the CXGGXR motif [49] , with an active-site cysteine in a glycine-rich loop (Fig. 6e , Supplementary Fig. 15 ). The crystal structure of Legionella pneumophila Lpg2838, a TrhO homolog, was solved by structural genomics (Supplementary Fig. 16 ) [50] . In the rhodanese domain, the active-site loop structure with the CTGGIR sequence (positions 200–205 in E. coli numbering) is formed by hydrogen bonds between T201 and R205 (corresponding to T178 and R182 in Supplementary Fig. 16). To characterize this motif, we constructed a series of E. coli trhO mutants in which C200, T201, G202, G203, R205, or C206 was mutated to alanine, and then examined their activities in vivo by complementation of the ∆ trhP /∆ trhO strain. The level of cmo 5 U34 in tRNA Val1 was partially restored by WT trhO (Fig. 6f ). For the trhO mutants, C200, T201, G203, and R205 were essential for trhO -mediated tRNA hydroxylation, whereas G202 and C206 were not (fig. 6f ). In the TrhO structure, a positively charged β-sheet is present near the active-site loop (Supplementary Fig. 16 ), providing a surface capable of recognizing tRNAs. The trhO mutants K112A and R114A, which lack positively charged residues on the β-sheet surface, hardly rescued or did not rescue cmo 5 U34 formation, respectively (Fig. 6f ), suggesting that this surface is required for trhO -mediated tRNA hydroxylation. In this study, we identified two independent pathways, mediated by trhP and trhO , involved in tRNA hydroxylation in the early steps of (m)cmo 5 U34 formation. We confirmed that (m)cmo 5 U34 was completely converted to unmodified U34 in a ∆ trhP /∆ trhO strain. This finding enabled us to analyze the physiological roles of (m)cmo 5 U34. This strain grew more slowly than a ∆ cmoB strain, which has ho 5 U34, confirming the physiological importance of the O5 oxygen atom of (m)cmo 5 U34. In addition, the ∆ trhP /∆ trhO strain exhibited severe growth defects and temperature-sensitive phenotypes when each of the tRNA genes ( serU , thrW , and proK ) responsible for G-ending codons was simultaneously deleted. These genetic interactions strongly indicate that (m)cmo 5 U34 plays a functional role in efficiently deciphering G-ending codons. The luciferase reporter assay revealed that decoding of UCG was significantly impaired in the ∆ trhP /∆ trhO strain relative to the ∆ cmoB strain in the absence of tRNA Ser2 , suggesting that the ho 5 UGA anticodon decodes the UCG codon more efficiently than the UGA anticodon. These observations demonstrate the direct involvement of the O5 oxygen of the xo 5 U34 modification in codon recognition in vivo. According to the crystal structure of the ribosome 30S subunit in complex with the anticodon-stem loop (ASL) of tRNA, cmo 5 U-G pairing forms Watson–Crick geometry (Supplementary Fig. 17 ), which is more stable than U-G wobble geometry due to the stacking interaction with the neighboring base pair (i.e., the second letters of codon and anticodon) [19] . The O5 oxygen of cmo 5 U34 makes a hydrogen bond with 2’ OH of U33 to pre-structure the ASL, presumably reducing entropic cost to base pair with any codons. In addition, the O5 oxygen may induce keto-to-enol tautomeric conversion of the uracil base to stabilize cmo 5 U-G pairing in Watson–Crick geometry. Moreover, because (m)cmo 5 U34 decodes G-ending codons more efficiently than ho 5 U34 [13] , [18] , the carboxymethyl group and terminal methylation of (m)cmo 5 U34 contribute further to efficient codon recognition. Structural analysis has shown that the carboxymethyl group of cmo 5 U34 forms a hydrogen bond with the O4 carbonyl oxygen of U in the first letter of the codon, implying that the cmo 5 U side chain is directly involved in codon recognition [19] . Because ho 5 U34 has a phenolic hydrogen, and the pK a value of O5 is 7.78 [51] , ho 5 U34 is ionized to some extent under neutral pH conditions. Thus, the carboxymethylation of cmo 5 U34 and methylation of mo 5 U34 might confer efficient codon recognition by suppressing the ionization of ho 5 U34. Our findings reveal that the TrhP-dependent pathway requires prephenate, whereas the TrhO-dependent pathway requires molecular oxygen. Thus, these two pathways are biochemically independent with respect to their requirement for metabolites. The existence of redundant and robust pathways for ho 5 U formation emphasizes that the xo 5 U34 modification is essential for bacteria to survive in a harsh environment. This is the unique instance of the RNA modification synthesized by two independent pathways in the same organism. According to phylogenetic distribution analysis in all domains of life (Supplementary Fig. 6 ), some organisms possess both trhP and trhO genes, whereas other organisms possess just one of them. Considering that anaerobes preceded aerobes in the early evolution on Earth, the trhP pathway might have been established in anaerobic bacteria before the trhO pathway arose, assuming that xo 5 U34 was present in such ancestral organisms. Presumably, the trhO pathway was acquired by aerobic bacteria after the O 2 concentration increased on Earth. The trhP pathway is required for anaerobic bacteria, whereas the trhP and trhO dual pathways are useful for organisms that live in both anaerobic and aerobic environments. TrhP is a peptidase U32-containing protein. Phylogenetic analysis has shown that peptidase U32-containing proteins can be classified into 12 subfamilies (Supplementary Fig. 1 ) [30] . We showed previously that three of these families include the RlhA proteins (RlhA1, RlhA2a, and RlhA2b) responsible for ho 5 C formation in 23S rRNA [30] . It is plausible that other subfamilies are also involved in hydroxylation of RNA or other biomolecules. Clostridia species harbor a member of the PepU32#1 family and trmR , but no homologs of trhO or trhP , implying that mo 5 U34 is present and that PepU32#1 family proteins are functional homologs of trhP in these species. Helicobacter pylori , a representative of the ε-proteobacteria, possesses a PepU32#2 family protein (HP0169), cmoA , and cmoB , but no homologs of trhO or trhP , indicating that cmo 5 U34 is present and suggesting that HP0169 is responsible for prephenate-dependent ho 5 U34 formation in this species. Intriguingly, HP0169 is required for gastric colonization by H. pylori [52] . Similarly, in Salmonella enterica , a trhP ortholog is associated with chicken macrophage infection [53] . Together, these findings suggest that xo 5 U34 contributes to bacterial infection and pathogenesis. We found that prephenate is required for trhP -dependent ho 5 U34 formation. Given that prephenate is also a substrate for cmo 5 U34 formation mediated by CmoA and CmoB [21] , it is a critical metabolite involved in the entire pathway of cmo 5 U34 biogenesis. Prephenate is generated from chorismate, which in turn is a common precursor of multiple metabolites, including aromatic amino acids, quinones, folate, and siderophores [47] . Thus, cmo 5 U34 modification might be tightly associated with the shikimate pathway and biogenesis of aromatic amino acids. The frequency of cmo 5 U34 might be regulated by the cellular concentration of prephenate under some environmental stress conditions. TrhP is a paralog of RlhA in the same family of peptidase U32-containing proteins. RlhA is responsible for prephenate-dependent ho 5 C2501 formation in E. coli 23S rRNA [30] , strongly implicating the involvement of the peptidase U32 motif in the C5-hydroxylation of pyrimidine base. Here, we showed that three conserved residues (E162, C170, and C177) in the motif of TrhP are essential for ho 5 U34 formation. Additionally, the corresponding residues (E161, C169, and C176) in RlhA were also required for ho 5 C2501 formation [30] , demonstrating that the peptidase U32 motif is directly involved in the hydroxylation of RNA. To date, we have no evidence that TrhP and RlhA directly catalyze the hydroxylation of RNA molecules. Given that RlhA is directly bound to the 50S subunit and its precursor in the cell, RlhA might be the hydroxylase responsible for ho 5 C2501 formation. By analogy, TrhP might be a hydroxylase for tRNA. Regarding the role of prephenate in ho 5 U34 formation, several possibilities should be considered. Prephenate might serve as an oxygen donor for ho 5 U34 formation, or alternatively as a coenzyme for the reaction. Moreover, we cannot exclude the possibility that unknown metabolites derived from prephenate are involved in ho 5 U34 formation. Further studies are necessary to elucidate the molecular mechanism underlying ho 5 U34 formation mediated by TrhP and prephenate. trhO homologs are present in many aerobes and facultative anaerobes, but not in obligate anaerobes such as Bacteroides , Clostridium , and Bifidobacterium . trhO homologs are distributed in a wide range of bacteria, including α-, β-, and γ-proteobacteria, Bacilli, actinobacteria, the FCB group, cyanobacteria, and a subset of phylum Tenericutes (Supplementary Fig. 6 ). Intriguingly, trhO homologs are also widely distributed in vertebrates and other eukaryotes. This finding suggests the presence of an xo 5 U-type modification in eukaryotes. We also showed that TrhO directly catalyzes oxygen-dependent ho 5 U34 formation. TrhO is related to rhodanese, which is involved in persulfide formation during detoxification of cyanide; however, the functions of most rhodanese family proteins remain unclear. In the context of RNA modifications, Tum1p is a rhodanese protein that mediates a persulfide sulfur for 2-thiouridine synthesis in eukaryotes [38] . Bacterial YbbB (also known as MnmH) is another rhodanese family protein responsible for biogenesis of 2-selenouridine (se 2 U) [54] and geranyl-2-thioudirine (ges 2 U) [55] . Mutation study of TrhO revealed that the active-site loop of the rhodanese domain is responsible for ho 5 U34 formation, suggesting that the rhodanese domain plays a critical role in hydroxylation of uracil base. Future studies should seek to clarify the mechanism by which rhodanese catalyzes this reaction. We now have a complete picture of xo 5 U34 formation in bacteria (Fig. 7 ). In the first step, U34 is redundantly hydroxylated by TrhP and TrhO to form ho 5 U34 in tRNAs responsible for decoding NYN codons. TrhP requires prephenate as a metabolite for ho 5 U34 formation, whereas TrhO uses a molecular oxygen for this purpose under aerobic conditions. In E. coli , TrhP is involved in ho 5 U34 formation of all six tRNA species, but has a preference for tRNA Leu3 and tRNA Pro3 , whereas TrhO mainly hydroxylates the other four species. CmoA employs prephenate and AdoMet to generate SCM-SAH, a metabolite used for carboxymethylation of ho 5 U34 to yield cmo 5 U34 catalyzed by CmoB. Four tRNAs (for Ala1, Ser1, Pro3, and Thr4) are further methylated by CmoM to yield mcmo 5 U34. mcmo 5 U34 in tRNA Ser1 is partially methylated by TrmL to yield mcmo 5 Um34 as a minor modification. In Gram-positive bacteria, including B. subtilis , ho 5 U34 is methylated by TrmR to yield mo 5 U34 instead of (m)cmo 5 U34. Fig. 7 Biogenesis of mcmo 5 U34 and derivatives. At the first step, U34 is redundantly hydroxylated by independent pathways mediated by TrhP and TrhO to form ho 5 U34 in tRNAs responsible for decoding NYN codons. TrhP requires prephenate as a metabolite for ho 5 U34 formation, whereas TrhO uses O 2 to hydroxylate U34 to form ho 5 U34 under aerobic conditions. CmoA synthesizes SCM-SAH from prephenate and AdoMet. CmoB uses SCM-SAH for carboxymethylation of ho 5 U34 to yield cmo 5 U34. Four tRNAs (for Ala1, Ser1, Pro3, and Thr4) are further methylated by CmoM to yield mcmo 5 U34. In Gram-positive bacteria, including B. subtilis , ho 5 U34 is methylated by TrmR to yield mo 5 U34 Full size image Strains and media A series of single-knockout strains of E. coli and their parent strain were obtained from the National BioResource Project (NBRP), National Institute of Genetics (NIG), Japan (Keio collection) [56] . Other knockout strains were generated by homologous recombination using λ-derived Red recombinase [57] with the chloramphenicol-resistance (Cm R ) or the kanamycin-resistance marker (Kan R ); all strains were selected with the appropriate antibiotics (20 µg per ml chloramphenicol or 50 µg per ml kanamycin). E. coli strains with multiple gene deletions were constructed by P1 transduction. The Kan R marker was removed by pCP20 transformation [56] . Genotyping of each construct was performed by colony PCR. A series of knockout strains [Δ yrrO (Δ trhP1 )::Em R , Δ yrrN (Δ trhP2 )::Em R , and Δ ybfQ (Δ trhO )::Em R ] and their parent strain [ B. subtilis 168 MGNA-A001 ( trpC2 )] were obtained from the NBRP, NIG, Japan [58] . To construct Δ yrrN /Δ yrrO , Δ yrrM , and Δ ybfQ /Δ yrrN /Δ yrrO strains, the Cm R cassette amplified from pDLK2 (courtesy of Akiko Soma, Chiba Univ.) was flanked by the 5’ and 3’ regions (~800 bps) of the target genes by ligation PCR, followed by transformation and selection with 5 µg per ml chloramphenicol. All constructs were confirmed by colony PCR. 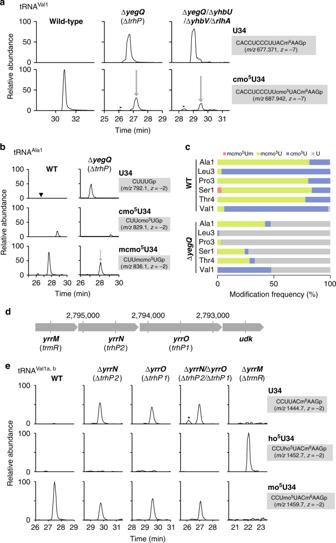Fig. 2 Identification oftrhPresponsible for tRNA hydroxylation.aMass-spectrometric shotgun analysis of total tRNAs inE. colistrains. Extracted ion chromatograms (XICs) show multiply charged negative ions of the anticodon-containing fragments of tRNAVal1with U34 (upper panels) and cmo5U34 (lower) in total tRNAs from wild-type (left), ∆yegQ(center), and ∆yegQ/∆yhbU/∆yhbV/∆rlhAstrains (right). Sequence,m/zvalue, and charge state of each fragment are shown on the right. Asterisks indicate nonspecific peaks with the samem/zvalues.bMass-spectrometric analysis of the wobble modification inE. colitRNAAla1isolated from WT (left panels) and ∆yegQ(right) strains. XICs show anticodon-containing fragments of tRNAAla1with U34 (top panels), cmo5U34 (middle panels), and mcmo5U34 (bottom panels). The cleavage sites of RNase T1are shown in Fig.1a. It is assumed that cmo5U detected in this tRNA was generated by artificial hydrolysis of mcmo5U during tRNA isolation13. The black arrowhead indicates a small peak corresponding to the U34-containing fragment detected in the WT.cModification frequencies of cmo5U derivatives at the wobble position of six tRNA species isolated from WT and ∆yegQstrains. Relative compositions of each modification were calculated from the peak area ratio of mass chromatograms of RNase T1digest fragments containing mcmo5Um (red), mcmo5U (green), cmo5U (blue), or U (gray) at the wobble position (Supplementary Fig.2)13. Source data are provided as a Source Data file.dGene organization of aB. subtilisoperon containingyrrM,yrrN, andyrrO. Genomic positions inB. subtilisare indicated. The new name for each gene is shown in parenthesis.eMass-spectrometric shotgun analysis of total tRNAs inB. subtilisstrains. XICs are shown of doubly charged negative ions of the anticodon-containing fragments of tRNAVal1a,bwith U34 (top panels), ho5U34 (middle panels), and mo5U34 (bottom panels) in total tRNA from wild-type (leftmost panels), ∆yrrN(left panels), ∆yrrO(middle panels), ∆yrrN/∆yrrO(right panels), and ∆yrrM(rightmost panels) strains All primers and strains used in this study are listed in Supplementary Data 3 and Supplementary Table 2 , respectively. M9 minimal medium with 0.4% glucose or LB medium, as well as the corresponding solid media containing 1.5% agar, were used for growth analysis of E. coli . MOPS medium with 20 amino acids (10 mM Ser, 0.8 mM Ala/Gly/Leu, 0.6 mM Gln/Glu/Val, 0.4 mM Arg/Asn/Ile/Lys/Phe/Pro/Thr, 0.2 mM His/Met/Tyr, and 0.1 mM Cys/Trp), five vitamins (0.02 mM thiamine hydrochloride, 0.02 mM calcium pantothenate, 0.02 mM 4-aminobenzoic acid, 0.02 mM 4-hydroxybenzoic acid, 0.02 mM 2,3-dihydroxybenzoic acid), 0.4% glucose, and appropriate antibiotics, in the presence or the absence of 1 mM prephenate (Sigma-Aldrich, St. Louis, MO, USA), was used to determine the metabolite required for the trhP pathway. Plasmid construction For the genetic rescue study, CDSs of trhP , trhO , and pheA with their 200 bp upstream sequences (including native promoter regions) were PCR-amplified from the E. coli BW25113 genome and cloned into pMW118 (Nippon Gene) to yield pMW-trhP, pMW-trhO, and pMW-pheA, respectively. pMW-pheA(CM), which lacks prephenate dehydratase activity due to the T278A mutation [48] , and a series of point mutants of pMW-trhP and pMW-trhO were constructed by QuikChange site-directed mutagenesis (Agilent Technology). For expression vectors of TrhO (YceA) and TrmR (YrrM), CDSs of trhO and trmR were PCR-amplified from genomic DNAs of E. coli BW25113 and B. subtilis 168, respectively, and cloned into pET21b (Novagen) to yield pET-trhO and pET-trmR. All constructs were confirmed by Sanger sequencing. All primers used in this study are listed in Supplementary Data 3 . RNA extraction and tRNA isolation Total RNA from each E. coli strain was extracted by phenol under acidic conditions [35] . The cells suspended in 1 × TE buffer [10 mM Tris (pH 8.0), 1 mM EDTA] was mixed with an equal volume of water-saturated phenol, followed by freeze and thaw twice and vigorous mixing for one hour at room temperature. The aqueous phase was separated by centrifugation, transferred to a new tube, washed with chloroform, and further purified using TRIzol reagent (Thermo Fisher Scientific, Waltham, MA, USA) and chloroform. RNA was recovered by 2-propanol precipitation. Individual tRNAs were isolated by reciprocal circulating chromatography (RCC) [42] using a series of DNA probes [13] (Supplementary Data 3 ). For RNA-MS shotgun analyses [13] , E. coli strains were cultured overnight, harvested, and resuspended in TE buffer to extract total RNA by TRIzol. The small RNA fraction was obtained as follows [13] . 50–250 μg of total RNA in 800 μl of 3 M NH 4 OAc (pH 5.3) was mixed with 640 μl (0.8 volume) of isopropanol at room temperature and centrifuged at 20,400× g for 10 min to precipitate long RNAs including rRNAs. The smaller RNA fraction was precipitated with ethanol from the supernatant. For RNA-MS shotgun analyses of B. subtilis tRNA modifications, the harvested cells were treated with 1 mg per ml lysozyme for 10 min on ice, and then subjected to TRIzol treatment to extract total RNA. Mass spectrometry of tRNA modifications Liquid chromatography–mass spectrometry (LC/MS) analyses of tRNA modification were conducted as follows [13] , [35] . For RNA fragment analyses of individual tRNAs and shotgun analyses, 1.25 pmol of tRNA or 50 ng of the small RNA fraction was digested with 50 units RNase T 1 (Thermo Scientific) in 20 mM NH 4 OAc (pH 5.3), followed by addition of an equal volume of 0.1 M triethylamine acetate (TEAA; pH 7.0). The RNase T 1 digests were subjected to the trap column for desalting and chromatographed by HiQ sil C18W-3 nanospray column (C18, 3μm, 120 Å pore size, ID 0.1 × 100 mm, KYA technologies) with solvent system consisted of 0.4 M 1,1,1,3,3,3-hexafluoro-2-propanol (HFIP) (pH 7.0) (solvent A) and 0.4 M HFIP (pH 7.0) in 50% methanol (solvent B) at a flow rate of 300 nl per min with a linear gradient of 5–100% B solvent over 35 min with a splitless nano HPLC system (DiNa, KYA Technologies). The eluent was ionized by ESI source and introduced into an ion trap-orbitrap hybrid mass spectrometer (LTQ Orbitrap XL, Thermo Fisher Scientific). Ions were scanned with a negative polarity mode over an m/z range of 600–2000 throughout the separation. XICs were plotted according to the theoretical m / z of each fragment (Supplementary Table 1 ). LC/MS nucleoside analysis was performed using Q Exactive Hybrid Quadrupole-Orbitrap Mass Spectrometer (Thermo Fisher Scientific) equipped with a Dionex UltiMate 3000 LC System (Thermo Fisher Scientific) essentially as described [13] , [59] . Twenty micrograms of the small RNA fraction were digested at 37 °C for 3 h in 60 µl of solution containing 20 mM trimethylamine-HCl (TMA-HCl) (pH 7.0), 0.05 U of nuclease P1, and 0.1 U of BAP. The digests mixed with acetonitrile (f.c. 90%) were chromatographed by ZIC-cHILIC column (3 μm particle size, 2.1 × 150 mm, Merck Millipore) with a guard column with the same resin (2.1 × 20 mm, Merck Millipore) using a solvent system consisted of 5 mM NH 4 OAc (pH 5.3) (solvent A) and acetonitrile (solvent B) at a flow rate of 100 μl min −1 in a multistep linear gradient; 90–40% B from 0 to 30 min, 40% B for 10 min, and then initialized to 90% B. The eluent was directly introduced into the ESI source and analyzed by mass spectrometer. Deprotonated nucleosides were scanned in a negative polarity mode over a m/z range of 110–700 throughout separation. Data were analyzed using Xcalibur software (Thermo Fisher Scientific). Basically, in negative mode of ESI, ionization efficiencies of the RNA fragments bearing the same sequence but different modification do not differ largely, because ESI ionization relies mainly on numbers of phosphate groups, not on type of base modifications [60] . Thus, we relatively quantified modification frequencies of RNA fragments with different chemical structures from their intensities of XICs. Luciferase reporter assay The dual-luciferase reporter assay [13] was performed as follows: knockout strains were transformed with pBAD-RFlucGCG, pBAD-RFlucUCG, or pBAD-RFlucGG. Each transformant was pre-cultivated at 37 °C in 2 ml LB medium containing 100 µg per ml ampicillin overnight. The preculture (1 ml) was inoculated to 2 ml of LB medium containing 100 µg per ml ampicillin and 100 µM arabinose to induce expression of the reporter. When the OD 600 reached to 0.3–0.7, 1 ml aliquot was centrifuged, and the pelleted cells were resuspended in 200 µl of lysis buffer [10 mM HEPES-KOH (pH 7.5), 100 mM NaCl, 10 mM MgCl 2 , 7 mM 2-mercaptoethanol, 400 µg per ml lysozyme]. Cell lysates were prepared by the freeze–thaw and cleared by centrifugation. The luciferase reporter assay was performed with 5 μl lysate using GloMax™ 96 Microplate Luminometer (Promega). The Fluc luminescence signal was normalized against the Rluc signal. Anaerobic cultivation WT and Δ trhP strains were precultured in a BioShaker G·BR-200 (TAITEC) at 37 °C with rotation at 60 rpm for 24 h in 10 ml of degassed LB medium in a 10 cm dish doubly packed in Ziploc (Asahi-Kasei, Japan) with one bag of AnaeroPack-Anaero (Mitsubishi Gas Chemical, Japan) and an oxygen indicator (OXY-1, JIKCO). The preculture (100 µl) was inoculated into 10 ml of degassed LB medium, sealed with an AnaeroPack-Anaero, incubated at room temperature for 1 h to deoxidize completely, and then cultivated at 37 °C overnight at 60 rpm. Metabolic labeling analysis using 18 O 2 18 O-containing mixed gas [20% 18 O 2 (97.5% 18 O 2 , 1% 17 O 2 , 1.5% 16 O 2 ), 80% N 2 ] was obtained commercially (Tatsuoka, Japan). The Δ cmoB /Δ trhP stain was precultured at 37˚C overnight in LB medium containing 50 µg per ml kanamycin. The preculture (1 ml) was inoculated into 100 ml of degassed LB medium containing 1 mM uridine and 50 µg/ml kanamycin packed in a PVDF air-sampling bag (As One, Japan). 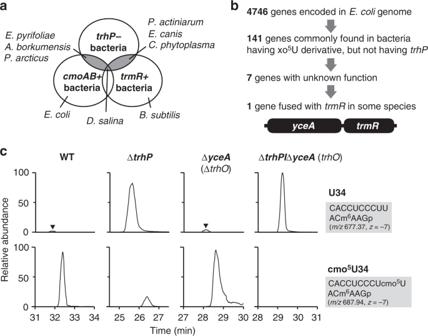Fig. 3 Identification oftrhOresponsible for tRNA hydroxylation.aVenn diagram depicts a group of organisms that havecmoABortrmRhomologs but notrhPhomologs.Erwinia pyrifoliae,Alcanivorax borkumensis, andPsychrobacter arcticusharborcmoABbut nottrhP;Pontibacter actiniarum,Ehrlichia canis, andCandidatus phytoplasmaharbortrmRbut nottrhP; andDactylococcopsis salinahas bothcmoABandtrmRbut nottrhP.bComparative genomics approach used to narrow down the candidate gene that bypasses ho5U34 biogenesis. InPhytophthora sojae,Phytophthora ramorum, andPhaeodatylum tricornutum,yceAandtrmRare fused as a single gene.cMass-spectrometric analysis of the wobble modification inE. colitRNAVal1isolated from WT (left panels), ∆trhP(middle left panels), ∆yceA(middle right panels), and ∆trhP/∆yceA(right panels) strains. XICs show anticodon-containing fragments of tRNAVal1with U34 (upper panels) and cmo5U34 (lower panels). Black arrowheads indicate peaks corresponding to U34-containing fragments detected in the WT and ∆yceA. Sequence,m/zvalue, and charge state of each fragment are shown on the right Inside air was carefully removed, and then replaced once with N 2 and twice with 18 O 2 mixed gas. The bag was capped and sealed with Parafilm (Bemis), and then cultured at 37 °C for 24 h at 100 rpm in a BioShaker G·BR-200 (TAITEC). Total RNA was extracted from the culture, digested into nucleosides, and analyzed by LC/MS as described above. Preparation of recombinant protein E. coli BL21(DE3) transformed with pET-trhO was cultured at 37 °C until OD 600 reached ~0.7, supplemented with 0.4% lactose, and further cultured at 16 °C for 32 h. The E. coli Rosetta(DE3) transformed with pET-trmR was cultured at 37 °C until OD 600 reached ~0.7, supplemented with 100 µM IPTG, and further cultivated at 37 °C for 4 h to induce overexpression. Cells were sonicated in lysis buffer for TrhO [50 mM HEPES-KOH (pH 7.5), 300 mM KCl, 10 mM MgCl 2 , 1 mM dithiothreitol (DTT), and 0.2 mM PMSF] or the lysis buffer for TrmR [50 mM HEPES-KOH (pH 7.5), 100 mM KCl, 10 mM MgCl 2 , 1 mM dithiothreitol (DTT), and 0.2 mM PMSF]. The recombinant proteins TrhO and TrmR were purified using a HisTrap column (GE Healthcare) with a linear gradient of imidazole (0–500 mM for TrhO, 25–500 mM for TrmR). Purified protein was dialyzed in the individual lysis buffer, supplemented with glycerol to a final concentration of 30%, and stored at −20 °C. In vitro reconstitution of tRNA modification For in vitro ho 5 U formation by TrhO, tRNA Ser1 transcript (10 pmol) and recombinant TrhO (10 or 100 pmol) were incubated at 37 °C for 1 h in a reaction mixture (10 µl) containing 25 mM Tris-HCl (pH 7.0), 300 mM NaCl, 1 mM MgCl 2 , and 10 mM 2-mercaptoethanol. The tRNA was extracted with acidic phenol/chloroform and precipitated with ethanol, followed by RNase T 1 digestion and RNA-MS analysis as described above. In vitro methylation of ho 5 U by TrmR was performed essentially as described [13] . E. coli tRNA Thr4 bearing ho 5 U34 was isolated from the Δ cmoB strain. The reaction mixture (10 µl) containing 10 pmol of tRNA Thr4 , 20 pmol of TrmR, 50 mM HEPES-KOH (pH 7.5), 100 mM KCl, 10 mM MgCl 2 , and 7 mM 2-mercaptoethanol was incubated at 37 °C for 1 h in the presence or absence of 1 mM AdoMet. Electrophoresis mobility shift assay EMSA was performed essentially as described [34] . Recombinant TrhO (0, 10, 20, 40, or 80 pmol) and in vitro transcribed tRNA Ala1 or tRNA Leu3 (20 pmol each) were incubated at 37 °C for 1 h in 10 µl of reaction mixture [50 mM HEPES-KOH (pH 7.5), 5 mM Mg(OAc) 2 , 100 mM KCl, 1 mM spermine, 1 mM DTT]. The mixtures were electrophoresed in 6% native polyacrylamide gel with running buffer [50 mM HEPES-KOH (pH 7.5), 5 mM Mg(OAc) 2 , and 1 mM DTT] in cold room. The gel was first stained with SYBR Safe (Thermo Fisher Scientific) to detect tRNA and then with Coomassie brilliant blue (Nacalai Tesque) to detect protein. Comparative genomics The comparative genomics approach used to identify the trhO ( yceA ) gene was performed with the IMG database [61] . The gene occurrence profile was used to select seven organisms in which cmoBA or yrrM homologs were present and trhP ( yegQ ) or trhP1/trhP2 homologs were absent: Ehrlichia canis str. Jake, Erwinia pyrifoliae DSM12163, Alcanivorax borkumensis SK2, Candidatus Phytoplasma asteris onion yellows OY-M, Pontibacter actiniarum sp. BAB1700, Dactylococcopsis salina PCC 8305, and Psychrobacter arcticus 273–4. Using the phylogenic profiler, 141 E. coli genes that are conserved in these seven organisms and B. subtilis were identified. According to the UniProt gene annotation, seven uncharacterized genes were picked as candidates. Phylogenetic analysis The phylogenetic tree of peptidase U32 (Supplementary Fig. 1 ) was generated as described [30] . Species names matched to proteins were retrieved from UniProt. The occurrence profiles of trhO , trhP , trhP1 , trhP2 , cmoA , cmoB , trmR , and cmoM homologs (Supplementary Fig. 6 ) were retrieved from GTOP [62] or the Interpro database [63] . 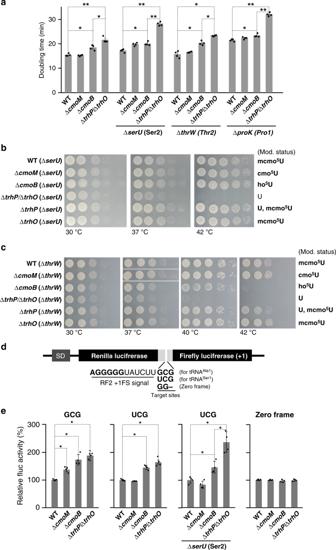Fig. 4 Phenotypes ofE. colistrains lacking tRNA hydroxylation.aGrowth rates ofE. colistrains with different wobble modifications. Doubling time of WT (mcmo5U34 for tRNASer1, tRNAThr4, and tRNAPro3), ∆cmoM(cmo5U34), ∆cmoB(ho5U34), and ∆trhP/∆trhO(U34) in the presence (left) or the absence of tRNA isodecoders at 37 °C in liquid LB medium: tRNASer2(middle left), tRNAThr2(middle right), or tRNAPro1(right). Individual data (dot plots) and their means ± SD (bar graph) are presented (n= 4). *P< 0.01; **P< 0.001 between two data series (Student’st-test, one-sided).bGrowth of WT, ∆cmoM, ∆cmoB, ∆trhP/∆trhO, ∆trhP, and ∆trhOstrains in the absence of tRNASer2(∆serU). The expected wobble modification status of each strain is shown on the right. Each strain was serially diluted (1:10), spotted onto LB agar plates, and cultivated for 11 h (30 °C), 8 h (37 °C) or 8 h (42 °C).cGrowth of WT, ∆cmoM, ∆cmoB, ∆trhP/∆trhO, ∆trhP, and ∆trhOstrains in the absence of tRNAThr2(∆thrW). The expected wobble modification of each strain is shown on the right. Each strain was serially diluted (1:10), spotted onto M9 minimum agar plates, and cultivated for 31 h (30 °C), 21 h (37 °C), 26 h (40 °C) or 31 h (42 °C).dSchematic of the reporter construct for the dual-luciferase assay, based on the RF2 recoding system. SD, Shine–Dalgarno sequence.Renillaand firefly luciferases were fused with a linker containing the +1 frameshift inductive signal of the RF2 recoding site. The frameshift target site was replaced with a GCG codon for tRNAAla1, a UCG codon for tRNASer1, or GG (zero frame) for the control.eRelative pausing activities at the frameshift site with a GCG codon (left), a UCG codon in the presence (middle left) or absence (middle right) of isodecoder tRNASer2, or zero frame (right) were calculated by normalizing Fluc activity vs. Rluc activity and further normalizing against the WT activity in each graph. Individual data and their means ± SD (n= 4) are presented. *P< 0.01 between two data series (Student’st-test, two-sided). All source data for Fig.4are provided as a Source Data file 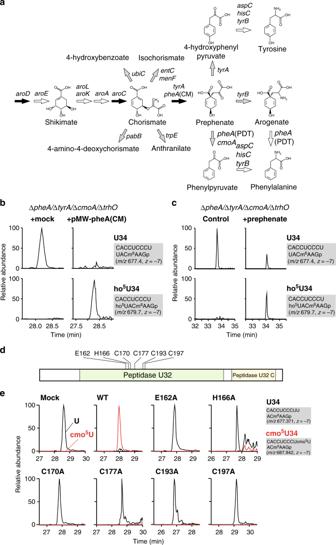Fig. 5 Characterization oftrhP-mediated tRNA hydroxylation.aA shikimate pathway and related metabolism. Chemical structures of metabolites and the responsible genes (italicized) at each step are shown. Two or three genes at each step indicate a redundant pathway [e.g., prephenate is redundantly synthesized from chorismate mediated bypheA(CM) andtyrA]. Black or gray arrows represent pathways indispensable or dispensable fortrhP-mediated ho5U34 formation, respectively (Supplementary Fig.9). White arrows represent pathways not examined in this study.bGenetic complementation of ho5U34 formation. Mass-spectrometric shotgun analysis of total tRNAs obtained from theE. coliΔpheA/ΔtyrA/ΔcmoA/ΔtrhOstrain transformed with a control plasmid (left panels) or pMW-pheA(CM) (right panels). XICs show multiply charged negative ions of anticodon-containing fragments of tRNAVal1with U34 (upper panels) and ho5U34 (lower panels). Sequence,m/zvalue, and charge state of each fragment are shown on the right.cMetabolic complementation of ho5U34 formation. Mass-spectrometric shotgun analysis of total tRNAs obtained from theE. coliΔpheA/ΔtyrA/ΔcmoA/ΔtrhOstrain cultured in the absence (left panels) or presence (right panels) of 1 mM prephenate. XICs show multiply charged negative ions of anticodon-containing fragments of tRNAVal1with U34 (upper panels) and ho5U34 (lower panels). Sequence,m/zvalue, and charge state of each fragment are shown on the right.dDomain organization ofE. coliTrhP, which contains Peptidase_U32 (PF01136) and Peptidase_U32_C (PF16325) domains. Six residues in the Peptidase_U32 domain that are essential for TrhP-mediated hydroxylation are indicated.eMutation study oftrhP. Mass-spectrometric shotgun analysis of total tRNA in theE. coli∆trhPstrain transformed with plasmid-encodedtrhPWT or mutants, as indicated. XICs show multiply charged negative ions of the anticodon-containing fragments of tRNAVal1with U34 (black lines) and cmo5U34 (red lines) in total tRNAs. Sequence,m/zvalue, and charge state of each fragment are shown on the right To generate the phylogenetic tree, 584 organisms that are registered in the databases we used, i.e., species listed in GTOP, phyloT, and Pfam, were selected. 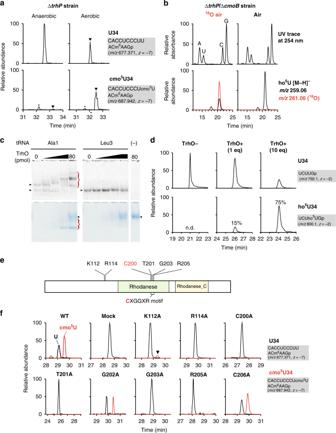Fig. 6 Characterization oftrhO-mediated tRNA hydroxylation.atrhO-mediated cmo5U formation takes place under aerobic conditions. Mass-spectrometric shotgun analysis of total tRNAs obtained fromE. coliΔtrhPstrain cultured under anaerobic (left panels) or aerobic (right panels) conditions. XICs show negative ions of the anticodon-containing fragments of tRNAVal1with U34 (upper panels) and cmo5U34 (lower panels). Arrowheads indicate target peaks, and asterisks indicate unspecific peaks.bMolecular O2is the metabolic source of the hydroxyl group of ho5U34 generated bytrhO. Mass-spectrometric nucleoside analyses of total RNAs obtained from theE. coli∆trhP/∆cmoBstrain cultured in mixed gas with 20%18O2(left panels) or in normal air (right panels). UV traces at 254 nm (upper panels) and XICs (lower panels) of deprotonated ho5U extracted from non-labeled (black line) or [18O]-labeled (red line) cells are shown.cTrhO interacts with tRNAAla1specifically. Electrophoretic mobility shift assay (EMSA) was performed to detect direct interaction between recombinant TrhO and tRNAAla1(left panels) or tRNALeu3(right panels) isolated fromE. coli. tRNAs and TrhO were stained with SYBR Safe (upper panels) and Coomassie brilliant blue (lower panels), respectively. TrhO–tRNA complexes are indicated by red traces. Arrowheads indicate unbound intact tRNAs and TrhO. Source data are provided as a Source Data file.dIn vitro reconstitution of ho5U34 with recombinant TrhO. RNase T1digests ofE. colitRNASer1transcripts (10 pmol) incubated with (10 pmol; 1 eq or 100 pmol; 10 eq) or without TrhO are subjected to RNA-MS. XICs show doubly charged negative ions of the anticodon-containing fragments of tRNA transcript with U34 (upper panels) and ho5U34 (lower panels). Frequencies of ho5U34 are indicated.eDomain organization ofE. coliTrhO bearing Rhodanese (PF00581) and Rhodanese_C (PF12368) domains. The CXGGXR motif and six residues mutated in this study are indicated.fMutation study oftrhO. Mass-spectrometric shotgun analysis of total tRNAs in theE. coliΔtrhP/ΔtrhOstrain transformed with plasmid-encodedtrhOWT or mutants, as indicated. XICs show multiply charged negative ions of the anticodon-containing fragments of tRNAVal1with U34 (black lines) and cmo5U34 (red lines) from total tRNA 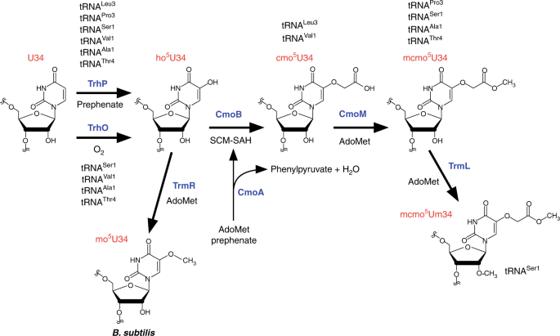Fig. 7 Biogenesis of mcmo5U34 and derivatives. At the first step, U34 is redundantly hydroxylated by independent pathways mediated by TrhP and TrhO to form ho5U34 in tRNAs responsible for decoding NYN codons. TrhP requires prephenate as a metabolite for ho5U34 formation, whereas TrhO uses O2to hydroxylate U34 to form ho5U34 under aerobic conditions. CmoA synthesizes SCM-SAH from prephenate and AdoMet. CmoB uses SCM-SAH for carboxymethylation of ho5U34 to yield cmo5U34. Four tRNAs (for Ala1, Ser1, Pro3, and Thr4) are further methylated by CmoM to yield mcmo5U34. In Gram-positive bacteria, includingB. subtilis, ho5U34 is methylated by TrmR to yield mo5U34 Reporting summary Further information on research design is available in the Nature Research Reporting Summary linked to this article.